Narrowband photodetection in the near-infrared with a plasmon-induced hot electron device In gratings, incident light can couple strongly to plasmons propagating through periodically spaced slits in a metal film, resulting in a strong, resonant absorption whose frequency is determined by the nanostructure periodicity. When a grating is patterned on a silicon substrate, the absorption response can be combined with plasmon-induced hot electron photocurrent generation. This yields a photodetector with a strongly resonant, narrowband photocurrent response in the infrared, limited at low frequencies by the Schottky barrier, not the bandgap of silicon. Here we report a grating-based hot electron device with significantly larger photocurrent responsivity than previously reported antenna-based geometries. The grating geometry also enables more than three times narrower spectral response than observed for nanoantenna-based devices. This approach opens up the possibility of plasmonic sensors with direct electrical readout, such as an on-chip surface plasmon resonance detector driven at a single wavelength. Plasmons—coherent oscillations of free electrons in metals—support intense electromagnetic field concentration, and provide the mechanism for harvesting light from free space and confining it to nanoscale volumes [1] , [2] . Interest in the properties of surface plasmons has recently expanded to encompass a broad range of technological applications, such as nonlinear optics [3] , [4] , metamaterials [5] , [6] , solar cell energy harvesting [7] , [8] , surface-enhanced sensing and spectroscopy [9] , [10] , and novel medical therapies [11] , [12] . These technologies rely, to varying degrees, on three key properties of plasmonic resonances: high field localization, resonant scattering and heat generation in nanoscale volumes. Another property of plasmons, their ability to generate hot electrons via plasmon decay at high efficiencies, has become a topic of rapidly increasing interest [13] , [14] , [15] . Recently several groups have reported tunable detection of light in metal–semiconductor devices by exploiting plasmon-induced hot electron generation [14] , [15] , [16] , [17] , [18] . In these devices, the incident electromagnetic radiation was coupled into surface plasmons by metallic nanoantennas patterned onto a semiconductor substrate. The nonradiative decay of the plasmons results in hot electrons that can transfer across the Schottky barrier at the metal–semiconductor interface and can be detected as a photocurrent [16] , [18] , [19] . This new type of Schottky photodetector enables a unique direct conversion of light captured by the antenna into an electrical signal: the tunability of the nanoantenna, such as its wavelength and polarization dependence, enables a straightforward ‘tailoring’ of the responsivity properties of the photodetector. The phenomenon of extraordinary optical transmission (EOT) on periodic metallic hole/slit structures provides another approach to light harvesting that could be useful for hot electron-based photodetection. Periodic slits form a grating [20] , [21] , which compensates for the momentum difference between propagating photons and plasmons, and enables the formation of surface plasmon waves capable of propagating on the metal surface [21] . In addition to propagation along on the upper surfaces, plasmons can also propagate through the slits of the grating. This phenomenon was first observed for metallic films with periodic hole arrays [22] . In EOT, plasmonic resonances enable far field transmission through perforations that can be significantly smaller than the minimum dimensions predicted using diffraction theory [23] . The same plasmon modes that give rise to EOT also give rise to hot electrons through nonradiative decay. By patterning a gold (Au) grating on a semiconducting substrate with an appropriately designed Schottky barrier at the interface, the hot electrons generated in the metallic structure should also give rise to a photocurrent response. Just as in the case of plasmonic nanoantennas, one would expect the optical response of the grating structure to be reflected in the electric current. This strategy has the additional advantage of a low-resistivity input face (the nanostructured metal film) that should enhance the transport properties of the device, including its responsivity. Here we report the first demonstration of a plasmonic grating-Schottky photodetector, which combines the resonant narrowband optical response of a grating structure with hot electron-enabled below bandgap photodetection. Device measurements showed a drastic increase in the responsivity and internal quantum efficiency (IQE) relative to earlier nanoantenna-based photodetectors, while simultaneously narrowing the spectral width of the photodetector response and preserving free-space coupling and polarization selectivity. The responsivity of this device (0.6 mA W −1 at zero bias voltage) is similar to responsivities reported in the literature for propagating plasmon sensors [24] . The IQE of this photodetector is ~0.2%, 20 times larger than the previously reported literature value of 0.01% for nanoantenna-based devices [16] . Unlike the previous reported devices mentioned, this responsivity maintains its narrowband full width at half maximum (FWHM) of nominally 54 meV, narrower by a factor of more than three compared with previously reported devices [16] , [18] . Using gratings also permits facile linear tuning of the responsivity peak over a broad wavelength regime in near-infrared (NIR), from 1,295 nm to 1,635 nm, enabling the use of conventional near-IR sources and also integration with other devices designed for this frequency range. Design of the grating hot electron device Our fabricated devices consist of high-purity Au gratings with different grating periods on a <100> n-type silicon wafer (500 μm thick, 1–10 Ωcm), with a 2-nm thick titanium adhesion layer ( Fig. 1a ). Although this thin titanium layer weakly damps the plasmon response [25] , it is crucial for both determining the Schottky barrier height and adhering the Au gratings to the silicon. We controlled the plasmonic response of the grating structure by varying three independent parameters: Au layer thickness ( T ), interslit distance ( D ) and slit width ( W ) ( Fig. 1a ). To investigate the dependence of the device properties on Au layer thickness, we fabricated three devices with T =93 nm, 170 nm and 200 nm ( Fig. 1b ), while keeping the slit width and interslit distance constant at 250 nm and 950 nm, respectively. Each grating covered a square measuring 12 × 12 μm. 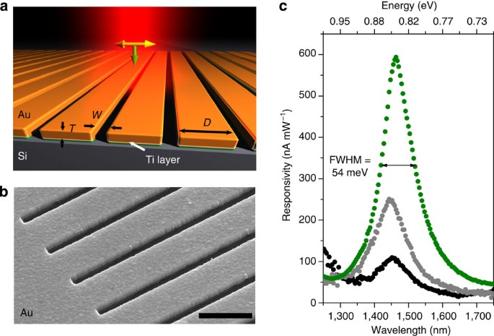Figure 1: Grating-Schottky photodetector. (a) Schematic of a gold grating on an n-type silicon substrate with a 2-nm Ti adhesion layer, oriented transverse to the laser polarization. For better visualization the thickness of Ti layer is exaggerated. Polarization of the incident laser and its k vector are represented in yellow and green arrows, respectively. (b) Scanning electron microscopy image of gold grating structure with grating thickness (T)=200 nm, interslit distance (D)=950 nm and slit width (W)=250 nm. For all structures the array measured 12 × 12 μm. The scale bar is 1 μm. (c) Photocurrent responsivities of grating-based photodetectors for three different gold layer thicknesses,T=93 nm (black), 170 nm (grey) and 200 nm (green), showing a strong intensity dependence on grating thickness. Figure 1: Grating-Schottky photodetector. ( a ) Schematic of a gold grating on an n-type silicon substrate with a 2-nm Ti adhesion layer, oriented transverse to the laser polarization. For better visualization the thickness of Ti layer is exaggerated. Polarization of the incident laser and its k vector are represented in yellow and green arrows, respectively. ( b ) Scanning electron microscopy image of gold grating structure with grating thickness ( T )=200 nm, interslit distance ( D )=950 nm and slit width ( W )=250 nm. For all structures the array measured 12 × 12 μm. The scale bar is 1 μm. ( c ) Photocurrent responsivities of grating-based photodetectors for three different gold layer thicknesses, T =93 nm (black), 170 nm (grey) and 200 nm (green), showing a strong intensity dependence on grating thickness. Full size image We obtained the photocurrent responsivities for three device thicknesses ( Fig. 1c ). For all three Au layer thicknesses, the spectral response shows a single, narrowband responsivity peak. The width of these peaks, which have a FWHM of 54±4 meV, is independent of grating thickness. For devices with a 200-nm thick Au layer, the peak responsivity increased by a factor of seven relative to the thinnest 93-nm grating, a trend reproduced in the calculated absorption spectra ( Supplementary Fig. S1 ). This significant increase illustrates the strong dependence of the absorption on Au film thickness, in a direct analogy with the known dependence of EOT on film thickness. Where EOT can enhance the transmission of light [22] , [26] , [27] , we can similarly exploit this effect to amplify plasmonic absorption at the metal–semiconductor interface [28] . The reflection and transmission spectra for these three thicknesses are provided in Supplementary Fig. S2 . The thickness dependence of the absorption cross-section of gratings is due to the interaction between propagating surface plasmons on the top and bottom surfaces of each Au pitch. In Fig. 2a , we schematically show the surface plasmons propagating on the upper and lower surfaces of the grating. These surface plasmons can interfere destructively or constructively with each other through the slits in the gratings. This interference allows us to minimize the destructive interference by using a specific thickness, which maximizes the amplitude of surface plasmon polariton decay—and hot electron generation—proximal to the interfacial region, increasing the photocurrent [29] . 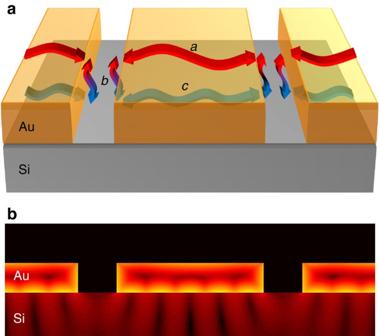Figure 2: Propagation of surface plasmons on gratings. (a) There are three forms of surface plasmon polaritons (SPPs) around each gold pitch:a, SPPs oscillating at the top surface of gratings;b, SPPs oscillating though the slits and;c, SPPs oscillating at the bottom surface of gratings at the Ti–Si Schottky interface. (b) Plasmonic heat absorption calculated by FDTD (shown with a logarithmic scale for clarity). Most of the hot electron generation occurs at the bottom surface of the gold layer. Figure 2: Propagation of surface plasmons on gratings. ( a ) There are three forms of surface plasmon polaritons (SPPs) around each gold pitch: a , SPPs oscillating at the top surface of gratings; b , SPPs oscillating though the slits and; c , SPPs oscillating at the bottom surface of gratings at the Ti–Si Schottky interface. ( b ) Plasmonic heat absorption calculated by FDTD (shown with a logarithmic scale for clarity). Most of the hot electron generation occurs at the bottom surface of the gold layer. Full size image The other reason for the high responsivity of grating-Schottky devices is the localization of absorption losses for gratings on silicon. The mean free path of the hot electrons in Au is ~35 nm [30] , [31] ; hot electrons generated in the Au further from the metal–semiconductor interface tend to lose energy through electron–electron scattering. Once the energy of a hot electron drops below the Schottky barrier height, transmission is unlikely to occur and the electron will reflect back into the Au without contributing to the photocurrent. To minimize these losses, the grating geometry has been designed to generate hot electrons primarily near the Schottky interface. This localized absorption can be seen in finite-difference time domain (FDTD) simulations of a representative structure with ( T, D, W )=(200, 950, 250) nm (olive curve, Fig. 1c ). Calculated absorption maps at the responsivity peak ( Fig. 2b , λ =1,460 nm) show that almost all the absorption occurs at the metal–semiconductor interface. Photodetector tuning For a given Au layer thickness, the grating resonance can be tuned through the NIR spectral regime by controlling the interslit distance ( D ) ( Fig. 3a ). Increasing D from 800 nm to 1,100 nm, in 50-nm increments, tuned the responsivity peak between 1,295 nm and 1,635 nm. For all seven gratings in Fig. 3 , the width W and thickness T were held constant at 250 nm and 200 nm, respectively. Wavelength selectivity was preserved when tuning the device over a broad spectral range, with all responsivity spectra exhibiting a peak FWHM of 53±6 meV. 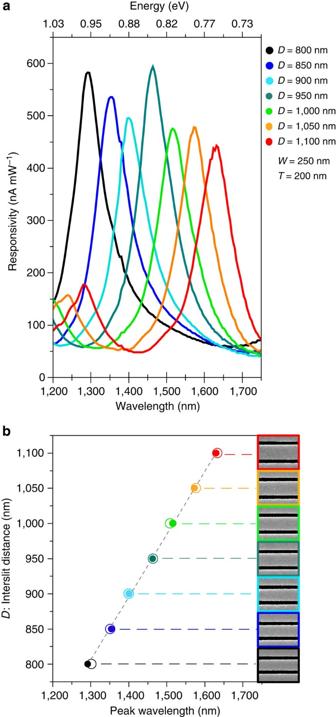Figure 3: Controlling the detection wavelength by tuning the interslit distance. (a) Responsivity peaks redshift with increasing grating interslit distance (D). ChangingDfrom 800 to 1,100 nm tuned the responsivity peak from 1,290 to 1,635 nm (T=200 nm,W=250 nm). The redshift in responsivity occurred with no change in FWHM. (b) FDTD (empty circles) and experimental data (filled circles) for the responsivity peak position in wavelength showing a linear dependence on interslit distance (grey dashed line). Images on the right show a representative top view scanning electron microscopy image of the grating for each corresponding responsivity peak. From bottom to top,Dincreases in 50-nm increments. Figure 3: Controlling the detection wavelength by tuning the interslit distance. ( a ) Responsivity peaks redshift with increasing grating interslit distance ( D ). Changing D from 800 to 1,100 nm tuned the responsivity peak from 1,290 to 1,635 nm ( T =200 nm, W =250 nm). The redshift in responsivity occurred with no change in FWHM. ( b ) FDTD (empty circles) and experimental data (filled circles) for the responsivity peak position in wavelength showing a linear dependence on interslit distance (grey dashed line). Images on the right show a representative top view scanning electron microscopy image of the grating for each corresponding responsivity peak. From bottom to top, D increases in 50-nm increments. Full size image The responsivity peaks exhibit a linear redshift with increasing interslit distance, D , which matches the spectra simulated using the FDTD method very well ( Fig. 3b ). The calculated responses were based on experimentally measured dimensions, and the optical constants of all materials used in our devices were parameterized using literature values with no adjustable parameters [32] , [33] , [34] . We presented the responsivity spectra for devices with the same interslit distances as mentioned in Fig. 3 , but different slit widths of 200 nm and 300 nm in Supplementary Fig. S3 . We can understand both the linear tunability of our photodetector and the lineshape by examining the surface charge distribution on a Au grating ( Fig. 4 ). A representative photocurrent spectrum, corresponding to a device with ( T, D, W )=(200, 1,100, 250) nm, shows two peaks at 1,635 nm and 1,285 nm, which we refer to as Mode i and Mode ii, respectively ( Fig. 4a ). A calculated absorption spectrum closely matches both the experimental linewidths and the relative peak amplitudes. For each of these modes we have calculated the surface charge density, where each blue and red region at the metal–silicon interface represents an anti-node of charge accumulation ( Fig. 4b ). For Mode i, surface charge oscillations at the metal–silicon interface have five anti-nodes, while the higher energy mode, Mode ii, has six anti-nodes. The number of anti-nodes defines the mode number of the standing surface plasmon. For a given mode number, increasing the interslit distance, D , linearly increases the wavelength of the standing wave at the metal–semiconductor interface proportionately, and therefore increases the wavelength of the responsivity peak with the same dependence. 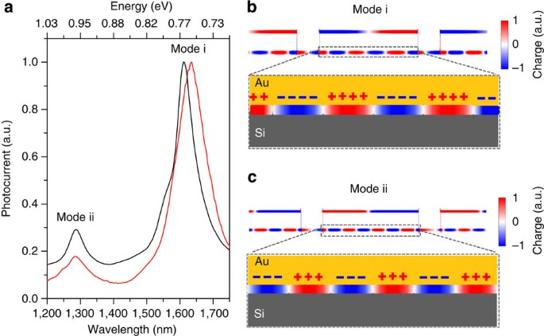Figure 4: Identification of the two modes in responsivity spectra. (a) FDTD (black curve) and experimental responsivity (red curve) spectra for the grating structure withT=200 nm,D=1,100 nm andW=250 nm. The corresponding responsivity curve has two modes: Mode i at the wavelength of 1,615 nm and Mode ii at the wavelength of 1,285 nm. (b) Surface charge plot at the metal–semiconductor interface at Mode i. (c) Surface charge plot at the metal–semiconductor interface at Mode ii. Figure 4: Identification of the two modes in responsivity spectra. ( a ) FDTD (black curve) and experimental responsivity (red curve) spectra for the grating structure with T =200 nm, D =1,100 nm and W =250 nm. The corresponding responsivity curve has two modes: Mode i at the wavelength of 1,615 nm and Mode ii at the wavelength of 1,285 nm. ( b ) Surface charge plot at the metal–semiconductor interface at Mode i. ( c ) Surface charge plot at the metal–semiconductor interface at Mode ii. Full size image One of the electrical limitations of these types of Schottky photodetectors is the Schottky barrier height at the metal–semiconductor interface. By fitting the I–V curve of our metal–semiconductor structure to the I–V characteristic of a typical Schottky diode, we extracted a barrier height of ~0.5 eV, similar to reported literature values of titanium and silicon Schottky barrier heights [35] . Controlled doping of the interfacial layer allows engineering of the Schottky barrier [36] , and could potentially be used to extend the effective detection range of these devices deep into the infrared, or increase device responsivities by raising the IQE. Visible-light detectors could also be designed by switching to higher-bandgap semiconductors than Si, such as TiO 2. Device responsivities can also be improved by increasing the Schottky contact area of the device, as shown recently by Scales et al . [37] . In summary, a narrowband, geometrically tunable photodetector in the NIR region has been demonstrated that combines the spectral properties of gratings with an electrical response based on plasmon-induced hot electron generation. The wavelength selectivity, linear tunability and high responsivity of the device make this type of photodetector useful for bridging the gap between optical and electrical systems. This unique type of device could have numerous applications requiring compact, wavelength-sensitive detection, such as chemical or bio-sensing, imaging and ranging, and communications systems. Device fabrication Our photodetectors were made by planar fabrication. The substrate was lightly doped n-type silicon coated with native oxide (1–10 Ωcm, <100> orientation). We deposited a 400-nm layer of photoresist (ZEP 520A, Zeon Corp.) by spin coating, and subsequently patterned using electron beam lithography. The samples were developed for 60 s in a 3:1 solution of ZED-ND50 (n-amyl acetate) to isopropanol. A reactive ion etch was used to strip the native oxide, and the samples were immediately transferred into an electron beam evaporator and coated with a 2-nm layer of titanium followed by a Au layer (devices used Au thicknesses of 93, 170 and 200 nm). Excess material was removed by liftoff in dimethylacetamide at 60 °C. The sample was then washed with isopropanol and dried with N 2 . Optical measurement techniques The photocurrent responsivities were obtained using a custom photocurrent microscope. Each device was illuminated at normal incidence by an ultrabroadband white-light laser (Fianium), with frequency selectivity achieved using an acousto-optical tunable filter (Crystal Tech.). For each frequency, the photocurrent was measured by modulating the laser source with a chopper and a lock-in amplifier (Signal Recovery, 7280DSP). The centre of each array was illuminated with the laser spot focused to ~3-μm FWHM, which eliminated contributions from the array edges (each grating was 12 × 12 μm). Measurements were taken with light polarized perpendicular to the slits; longitudinally polarized light does not couple to grating modes [38] and gave no measureable photocurrent. FDTD simulations FDTD simulations were done in two dimensions using the experimental dielectric function from Johnson and Christy for the Au material. The size of each modelled grating was 12 μm to match the fabricated devices. The incident beam was an s-polarized free-space electromagnetic wave with transverse polarization of the electric field to the orientation of slits. The beam had a Gaussian profile with a FWHM of 3 μm, which was approximately the same as the experimentally used spot size. Absorption spectra were calculated by integrating the total absorption within each simulated grating array. IQE calculation IQE was calculated according to IQE=100 × ( I p / q )/( P ab / hν ) in percentage, where I p is the photocurrent, q is the electron charge, P ab is the power of absorbed light and hν is the photon energy. How to cite this article: Sobhani, A. et al . Narrowband photodetection in the near-infrared with a plasmon-induced hot electron device. Nat. Commun. 4:1643 doi: 10.1038/ncomms2642 (2013).